Spin waves and magnetic exchange interactions in insulating Rb0.89Fe1.58Se2 The parent compounds of iron pnictide superconductors are bad metals with a collinear antiferromagnetic structure and Néel temperatures below 220 K. Although alkaline iron selenide A y Fe 1.6+ x Se 2 ( A =K, Rb, Cs) superconductors are isostructural with iron pnictides, in the vicinity of the undoped limit they are insulators, forming a block antiferromagnetic order and having Néel temperatures of roughly 500 K. Here we show that the spin waves of the insulating antiferromagnet Rb 0.89 Fe 1.58 Se 2 can be accurately described by a local moment Heisenberg Hamiltonian. A fitting analysis of the spin wave spectra reveals that the next-nearest neighbour couplings in Rb 0.89 Fe 1.58 Se 2 , (Ba,Ca,Sr)Fe 2 As 2 , and Fe 1.05 Te are of similar magnitude. Our results suggest a common origin for the magnetism of all the Fe-based superconductors, despite having different ground states and antiferromagnetic orderings. Soon after the discovery of superconductivity in iron pnictides [1] , calculations and experiments found that the electronic band structures of these materials are composed of hole and electron Fermi pockets near the Γ(0,0) and M(1,0)/M(0,1) points, respectively [2] . As a consequence, sign-reversed quasiparticle excitations between the hole and electron pockets can induce s ± -wave superconductivity, giving rise to a neutron spin resonance at the in-plane antiferromagnetic (AF) wave vector Q =(1,0) ( Fig. 1 ) [3] , [4] , [5] , [6] , [7] . These results suggest that the s ± -wave electron pairing mechanism is a leading candidate for the microscopic origin of superconductivity in all iron-based superconductors [2] . 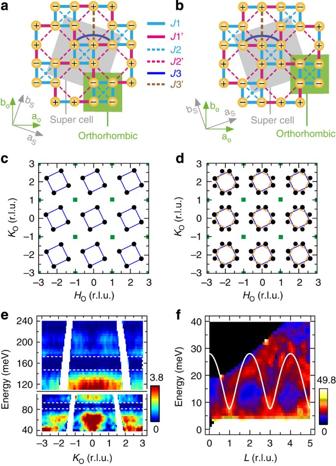Figure 1: The antiferromagnetic spin structure andc-axis spin waves of the insulating Rb0.89Fe1.58Se2. Our neutron scattering experiments were carried out on the ARCS chopper spectrometer at the Spallation Neutron Source, Oak Ridge National Laboratory. We co-aligned 2.7 g of single crystals grown by self-flux (with mosaic of ~6°). The incident beam energies wereEi=80,140,250,440 meV, and mostly withEiparallel to thec-axis. Spin wave intensities were normalized to absolute units using a vanadium standard (with 50% error). We define the wave vectorQat (qx,qy,qz) as (Ho;Ko;Lo)=(qxao,/2π;qyao/2π;qzco/2π) r.l.u., whereao=5.65 andco=14.46 Å are the orthorhombic cell lattice parameters. The AF spin structures are shown for (a) left and (b) right chirality. The √5×√5 superlattice structure is marked as grey with lattice parameteras=8.933 Å. The orthorhombic lattice cell is shaded green. The effective nearest neighbour, next nearest neighbour, next-next nearest neighbour exchange couplings are marked asJ1/J′1,J2/J′2, andJ3/J′3, respectively. (c) The [Ho, Ko] reciprocal space with the expected AF Bragg peaks from the left chirality. The green squares show nuclear Bragg peak positions. (d) Expected Bragg peaks for both chiralities. (e) Spin waves projected onto theKo-Eplane withHointegration from −2 to −1. The scattering were measured withEi=440,250 meV for top and bottom panels, respectively. (f)c-axis spin wave dispersion projected on theL–Eplane withHointegration from 0.5 to 0.7 andKintegration from 0 to 0.4. The solid line is the calculatedc-axis dispersion using effective exchange couplings discussed in the main text. Figure 1: The antiferromagnetic spin structure and c -axis spin waves of the insulating Rb 0.89 Fe 1.58 Se 2 . Our neutron scattering experiments were carried out on the ARCS chopper spectrometer at the Spallation Neutron Source, Oak Ridge National Laboratory. We co-aligned 2.7 g of single crystals grown by self-flux (with mosaic of ~6°). The incident beam energies were E i =80,140,250,440 meV, and mostly with E i parallel to the c -axis. Spin wave intensities were normalized to absolute units using a vanadium standard (with 50% error). We define the wave vector Q at ( q x , q y , q z ) as ( H o ; K o ; L o )=( q x a o ,/2 π ; q y a o /2 π ; q z c o /2 π ) r.l.u., where a o =5.65 and c o =14.46 Å are the orthorhombic cell lattice parameters. The AF spin structures are shown for ( a ) left and ( b ) right chirality. The √5×√5 superlattice structure is marked as grey with lattice parameter a s =8.933 Å. The orthorhombic lattice cell is shaded green. The effective nearest neighbour, next nearest neighbour, next-next nearest neighbour exchange couplings are marked as J 1 / J′ 1 , J 2 / J′ 2 , and J 3 / J′ 3 , respectively. ( c ) The [ H o , K o ] reciprocal space with the expected AF Bragg peaks from the left chirality. The green squares show nuclear Bragg peak positions. ( d ) Expected Bragg peaks for both chiralities. ( e ) Spin waves projected onto the K o - E plane with H o integration from −2 to −1. The scattering were measured with E i =440,250 meV for top and bottom panels, respectively. ( f ) c -axis spin wave dispersion projected on the L – E plane with H o integration from 0.5 to 0.7 and K integration from 0 to 0.4. The solid line is the calculated c -axis dispersion using effective exchange couplings discussed in the main text. Full size image The recent discovery of alkaline iron selenide A Fe 1.6+ x Se 2 ( A =K, Rb, Cs) superconductors [8] , [9] , [10] , [11] , [12] has generated considerable new excitement in the condensed matter physics community because superconductivity in these materials may have a different origin from the sign-reversed s -wave electron-pairing mechanism [13] , [14] , [15] , [16] . Although A Fe 1.6+ x Se 2 are isostructural with the metallic AF iron pnictides such as (Ba,Ca,Sr)Fe 2 As 2 (ref. 3 ), they are insulators near x =0 (refs 10 , 11 , 12 ) and form a √5×√5 block AF structure with Fe vacancy order ( Fig. 1a ) completely different from the iron pnictides [17] , [18] , [19] , [20] , [21] , [22] . If sign-reversed electron-hole pocket excitations between Γ(0,0) and M(1,0)/M(0,1) points are necessary for superconductivity, superconductivity in alkaline iron selenides should have a different microscopic origin because angle-resolved photoemission experiment measurements on these materials reveal only electron Fermi surfaces at M(1,0)/M(0,1) points and no hole Fermi pockets at Γ(0,0) point [13] , [14] , [15] . On the other hand, if AF spin excitations are responsible for superconductivity in Fe-based superconductors [23] , one would expect that spin waves in the parent compounds of different classes of Fe-based superconductors have a similar energy scale despite dramatically different transport and magnetic properties. Previous work on spin waves of (Ba,Ca,Sr)Fe 2 As 2 (refs 24 , 25 , 26 ) and Fe 1.05 Te (ref. 27 ) suggests that the overall magnetic spectra can only be described by considering both the local and itinerant electrons, and the next-nearest neighbour (NNN) exchange couplings in these materials are similar. Because the insulating A Fe 1.6+ x Se 2 has completely different magnetic structure, Néel temperatures, and static-ordered moments ( Fig. 1 ) from those of (Ba,Ca,Sr)Fe 2 As 2 and Fe 1.05 Te (ref. 3 ), it is important to determine whether spin waves in this material have an overall energy scale similar to other iron-based materials. Here we use inelastic neutron scattering to map out spin waves in the AF-insulating Rb 0.89 Fe 1.58 Se 2 . We find that although Rb 0.89 Fe 1.58 Se 2 has a Néel temperature ( T N =475 K) much higher than that of the iron pnictides ( T N ≤220 K) [3] , spin waves for both classes of materials have similar zone boundary energies [24] , [25] , [26] . However, although itinerant electrons must be considered to understand spin wave properties in the AF iron pnictides [24] , [25] , [26] , a local moment Heisenberg Hamiltonian can effectively describe the entire spin wave spectra of the AF Rb 0.89 Fe 1.58 Se 2 . A comparison of the Heisenberg-Hamiltonian-fitted effective exchange couplings in Rb 0.89 Fe 1.58 Se 2 , (Ba,Ca,Sr)Fe 2 As 2 (refs 24 , 25 , 26 ), and iron chalcogenide Fe 1.05 Te (ref. 27 ) reveals that their NNN exchange couplings are similar. Therefore, the NNN magnetic interactions in the AF alkaline iron selenides, iron arsenides and iron tellurides, which are robust against the change of electronic band structures, must mainly stem from the superexchange interactions mediated by As/Se(Te), and may have a key role in the magnetism of Fe-based superconductors. The AF spin structure, reciprocal space, and spin waves Before carrying out inelastic neutron scattering studies of spin waves in the insulating Rb 0. 89 Fe 1.58 Se 2 , we used polarized neutron-diffraction measurements to confirm the previously proposed Fe 4 block AF checkerboard structure ( Fig. 1a ) [19] , [22] . As the ferromagnetic (FM) Fe 4 block in the √5×√5 superlattice unit cell can have either left or right chirality ( Figs 1a,b ), one expects to observe four AF Bragg peaks stemming from each of the chiralities. Fig. 1c shows the expected AF peaks from the left chirality in reciprocal space using the orthorhombic unit cell similar to that of iron pnictides [24] , [25] , [26] , where they occur at ( H o ,K o ,L o )=(0.2+ m ,0.6+ n,L o ); (−0.2+ m ,−0.6+ n;L o ); (0.6+ m ,−0.2+ n,L o ); (−0.6+ m ,0.2+ n,L o ); ( m,n =±2,±4,..., and L o =±1, ±3,...). Considering both chiralities for the AF order, there are eight Bragg peaks at wave vectors H o ,K o ,L o )=(±0.2+ m ,± 0.6+ n,L o ) and ( H o ,K o ,L o )=(±0.6+ m ,±0.2+ n,L o ) from the block AF checkerboard structure ( Fig. 1d ), where the odd values of L o indicate AF coupling along the c -axis direction [19] , [20] , [21] , [22] . Therefore, acoustic spin waves in the AF-ordered phase of Rb 0.89 Fe 1.58 Se 2 should stem from these eight Bragg peaks. Before mapping out the wave vector dependence of spin waves in Rb 0.89 Fe 1.58 Se 2 , we first determine their overall energy bandwidth and the effective c -axis coupling. Figure 1e shows the background-subtracted scattering projected in the wave vector ( Q =[−1.5, K o ]) and energy plane. One can see three clear plumes of scattering arising from the in-plane AF zone centres Q =(0,−2),(0,0), and (0,2) r.l.u. With increasing energy, spin waves are gapped at energies between 75 and 95 meV (the bottom panel of Fig. 1e ) and between 150 and 170 meV (the top panel of Fig. 1e ). The zone boundary spin wave energies are around 220 meV (the top panel of Fig. 1e ). Therefore, in spite of the large differences in Néel temperatures and AF structures of Rb 0.76 Fe 1.6 Se 2 ( T N =475 K) [19] , [20] , [21] , [22] , (Ba,Ca,Sr)Fe 2 As 2 ( T N ≤220 K) [24] , [25] , [26] , and Fe 1.05 Te ( T N ~70 K) [27] , their zone boundary spin wave energies are rather similar. To estimate the AF coupling strength along the c -axis, we show in Figure 1f spin waves projected in the wave vector Q =[0.6,0.2, L o ] and energy space. One can see clear dispersive spin waves stemming from AF positions L o =1,3,5 that reach the zone boundary energy near 30 meV. 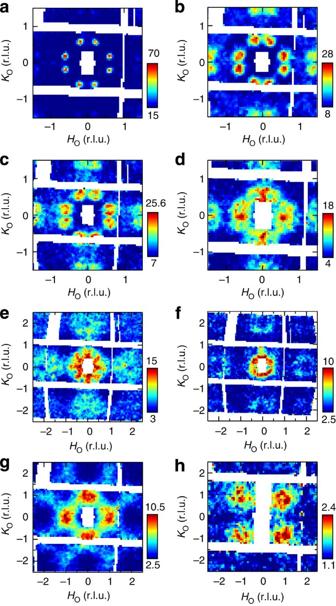Figure 2: Wave vector dependence of spin wave excitations at different energies for Rb0.89Fe1.58Se2at 10 K. Spin wave excitations in the [Ho, Ko] scattering plane at energies (a)E=10±2; (b)E=26±2; (c)E=30±2; (d)E=45±3; (e)E=55±3; (f)E=70±3; (g)E=110±10; and (h)E=200±20 meV. (a–c), (d–f),(g,h) were obtained withEi=80, 140, 250, and 440 meV, respectively, along thec-axis. The vertical colour bars indicate intensity scale in mbarns per sr per meV per f.u. Evolution of spin waves To see the evolution of spin waves with increasing energy, we show in Figure 2 the two-dimensional constant-energy ( E ) images of spin waves in the [ H o , K o ] plane, for various incident beam energies ( E i ). From their c -axis dispersion ( Fig. 1f ), we know that spin waves in Rb 0.89 Fe 1.58 Se 2 are three-dimensional, similar to those in (Ba,Ca,Sr)Fe 2 As 2 (refs 24 , 25 , 26 ), and centre at AF wave vectors Q AF =( H o , K o , L o )=(±0.2+ m ,±0.6+ n,L )/(±0.6+ m ,±0.2+ n,L ) with L o =±1,±3,... r.l.u. For an energy transfer of E =10±2 meV (above the anisotropy gap of E =8 meV, Methods; Supplementary Fig. S1 ), spin waves are peaked at the expected eight AF Bragg positions Q AF around Q =(0,0,±1) r.l.u. as shown in Figure 2a . On increasing energies to E =26±2 ( Fig. 2b ) and 30±2 meV ( Fig. 2c ), spin waves from the two chiralities centred around the Q AF positions become apparent and increase in size with increasing energy. The two spin wave rings from the left and right AF chiralities ( Figs 1a–d ) meet near E =45±3 meV ( Fig. 2d ). At E =55±3 meV, the overlapping spin waves from both AF chiralities still form rings around the Q AF positions ( Fig. 2e ). The spin waves have evolved into broad rings centred around ( H o , K o , L o )=(± m ,± n,L o ) at E =70±3 meV as shown in Figure 2f , just before disappearing into the 75≤ E ≤95 meV spin gap ( Fig. 1e ). On re-emerging from the spin gap at an energy transfer of 110±10 meV, the spin waves form transversely elongated ellipses centred at the wave vectors Q =(±1,0)/(0,±1) ( Fig. 2g ), identical to the AF ordering wave vector of (Ba,Ca,Sr)Fe 2 As 2 (refs 24 , 25 , 26 ). Finally, at E =200±20 meV, an energy well above the 150 ≤ E ≤ 170 meV spin gap, the spin waves move into wave vectors Q =(±1,±1) ( Fig. 2h ), almost identical to the zone boundary spin waves for BaFe 2 As 2 (ref. 24 ) and Fe 1.05 Te (ref. 27 ). Figure 2: Wave vector dependence of spin wave excitations at different energies for Rb 0.89 Fe 1.58 Se 2 at 10 K. Spin wave excitations in the [ H o , K o ] scattering plane at energies ( a ) E =10±2; ( b ) E =26±2; ( c ) E =30±2; ( d ) E =45±3; ( e ) E =55±3; ( f ) E =70±3; ( g ) E =110±10; and ( h ) E =200±20 meV. ( a–c ), ( d – f ),( g , h ) were obtained with E i =80, 140, 250, and 440 meV, respectively, along the c -axis. The vertical colour bars indicate intensity scale in mbarns per sr per meV per f.u. Full size image Heisenberg Hamiltonian We use a local moment Heisenberg Hamiltonian with the effective nearest (NN or J 1 , J′ 1 ), next-nearest (NNN or J 2 , J′ 2 ), and next-next-nearest neighbour (NNNN or J 3 , J′ 3 ) magnetic exchange couplings ( Fig. 1a ) to fit the observed spin-wave spectra [28] , [29] , [30] , [31] , [32] . To account for the ~8 meV low-energy spin gap (Methods), we add a spin anisotropy term J s to align spins along the c -axis ( Supplementary Eqs S1–S7 ). There are eight spins in each magnetic unit cell ( Fig. 1a,b ); therefore, we should have four doubly-degenerate spin wave bands in the Brillouin zone. From Figures 1 and 2 , we see that spin waves exist in three separate energy ranges: the lowest branch starts from ~9 meV to ~70 meV, the second one from ~80 meV to ~140 meV, and the third branch from ~180 meV to ~230 meV. The high quality spin wave data allows us to place quantitative constraints on effective exchange couplings in the Heisenberg Hamiltonian ( Supplementary Eqs. S15–S23 ). While the low-energy spin waves between ~9 meV and ~70 meV are acoustic modes arising mostly from AF interactions of the FM-blocked spins, the two other branches of excitations are optical spin waves associated with exchange interactions of iron spins within the FM blocks [29] , [30] , [31] , [32] . We have attempted, but failed, to fit the entire spin wave spectra using only the effective NN and NNN exchange-coupling Heisenberg Hamiltonian ( Fig. 3 ; Supplementary Figs S1–S4 ). For spin wave fits that include the NNNN exchange coupling J 3 , we find that the low energy spin wave band (acoustic band) depends mainly on J′ 1 , J′ 2 , J 3 , and J c (the effective c -axis exchange coupling), but not J 1 and J 2 . The second band depends on the J 2 heavily and the top band is mainly determined by J 1 . 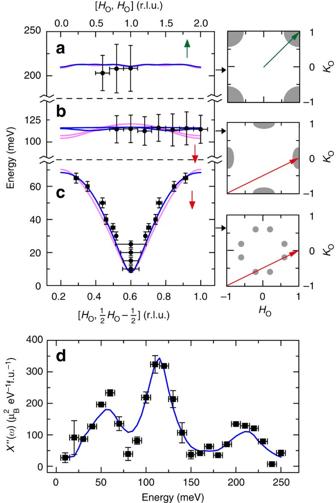Figure 3: Spin wave dispersions of Rb0.89Fe1.58Se2and fits using the Heisenberg Hamiltonian. Spin wave dispersions obtained by cutting along high symmetry directions marked in the right panels for (a) highest energy optical-energy band; (b) medium-energy optical energy band; and (c) acoustic spin wave mode. The blue solid lines show fits withJ3>0, while the pink solid lines are fits withJ3=0. (d) The energy dependence of the local susceptibility and our model calculation of the local susceptibility. The vertical error bars indicate the statistical errors of one standard deviation. Figure 3: Spin wave dispersions of Rb 0.89 Fe 1.58 Se 2 and fits using the Heisenberg Hamiltonian. Spin wave dispersions obtained by cutting along high symmetry directions marked in the right panels for ( a ) highest energy optical-energy band; ( b ) medium-energy optical energy band; and ( c ) acoustic spin wave mode. The blue solid lines show fits with J 3 >0, while the pink solid lines are fits with J 3 =0. ( d ) The energy dependence of the local susceptibility and our model calculation of the local susceptibility. The vertical error bars indicate the statistical errors of one standard deviation. Full size image For simplicity, we consider each FM block with four aligned spins as a net spin S eff . They interact with each other antiferromagnetically (via J eff ) to form a cuprates like AF spin structure. There is one spin wave band for this effective block-spin Heisenberg model, which has an analytical form for spin wave dispersion ( Supplementary Eq. S15 ). By comparing the J eff Heisenberg Hamiltonian with those of the J 1 - J′ 1 - J 2 - J′ 2 - J 3 - J′ 3 model, we find that spin waves in the first band can be approximately described by the J eff Heisenberg Hamiltonian, where J eff S eff =( J′ 1 +2 J′ 2 +2 J 3 ) S /4 is ~17 meV. This suggests that the low energy band is mainly determined by J′ 1 , J′ 2 , J 3 , and J c . Physically, the lowest energy band corresponds to the block spin waves where the four spins fluctuate in phase and resemble a single spin. Only at high energies, the relative motions within the blocks can be excited, which correspond to the two high-energy optical modes. Thus, the high-energy bands are basically determined by the intra-block couplings J 1 and J 2 . To quantitatively determine the spin wave dispersion, we determined the measured dispersion from a series of high-symmetry scans through the ( H o , H o , L o ) and ( H o ,1/2 H o −1/2, L ) directions, where L o was integrated to improve counting statistics. Fig. 3a–c summarize the dispersion of spin waves along the marked directions on the right panels. For the low-energy acoustic mode, we find a spin anisotropy gap below 8 meV and counter propagating spin waves for energies above 30 meV ( Fig. 3c ). The two high-energy optical spin wave modes are essentially dispersionless. The blue and pink solid lines show Heisenberg Hamiltonian fits to the dispersion curves with and without J 3 . The final fitted effective magnetic exchange couplings for spin wave dispersions are SJ 1 =−36±2, SJ′ 1 =15±8, SJ 2 =12±2, SJ′ 2 =16±5, SJ 3 =9±5, J′ 3 =0, SJ c =1.4±0.2, and SJ s =0.44±0.1 meV ( Supplementary Figs S1–S5 for fits with other parameters). Figure 3d shows the energy dependence of the observed local susceptibility [33] and our calculation using the fitted parameters. We see that the calculated local susceptibility agrees quite well with the data. 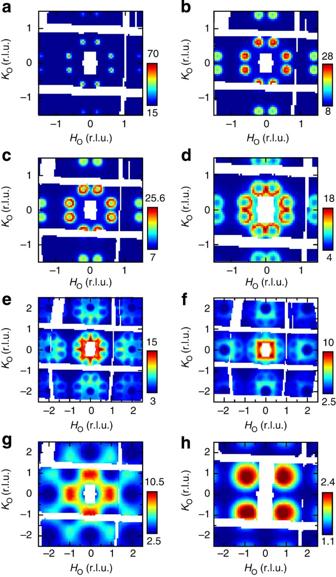Figure 4: Calculated energy dependence of the spin waves. The wave vector dependence of the spin waves in the [Ho, Ko] scattering in absolute units for energies of (a)E=10±2; (b)E=26±2; (c)E=30±2; (d)E=45±3; (e)E=55±3; (f)E=70±3; (g)E=110±10; and (h)E=200±20 meV. The instrumental resolution is convoluted with the Heisenberg Hamiltonian. To further compare the data in Figure 2 with calculated spin waves using fitted effective exchange couplings, we show in Figure 4 the two-dimensional spin wave projections in the [ H o ,K o ] plane convoluted with instrumental resolution. The calculated spin wave spectra capture all essential features in the data. Figure 4: Calculated energy dependence of the spin waves. The wave vector dependence of the spin waves in the [ H o , K o ] scattering in absolute units for energies of ( a ) E =10±2; ( b ) E =26±2; ( c ) E =30±2; ( d ) E =45±3; ( e ) E =55±3; ( f ) E =70±3; ( g ) E =110±10; and ( h ) E =200±20 meV. The instrumental resolution is convoluted with the Heisenberg Hamiltonian. Full size image For a Heisenberg model with spin S , the total moment sum rule stipulates M 0 =( g μ B ) 2 S ( S +1) (ref. 34 ). For irons in the 3 d 6 electronic state, the maximum possible moment is gS =4 μ B /Fe for g =2, giving M 0 =24 μ 2 B /Fe. On the basis of absolute spin wave intensity measurements in Figure 3d , the sum of the fluctuating moments within the Brillouin zone ( Supplementary Fig. S5 ) below ~250 meV is ‹ m 2 ›~16±3 μ B 2 /Fe. If we assume that the ordered moment is on the order of ~3 μ B /Fe (refs 19 , 20 , 21 ), we see that the total moment sum rule is exhausted for magnetic scattering at energies below 250 meV. Therefore, spin waves in insulating Rb 0.76 Fe 1.63 Se 2 can be regarded as a classic local moment system where a Heisenberg Hamiltonian is an appropriate description of spin wave spectra. For comparison, we note that the sum of the fluctuating local moments throughout the Brillouin zone for AF metallic BaFe 2 As 2 (ref. 24 ) and superconducting BaFe 1.9 Ni 0.1 As 2 (ref. 35 ) are ‹ m 2 ›=3.17±0.16 and 3.2±0.16 μ B 2 per Fe(Ni), respectively (M.S. Liu et al ., unpublished results). Because ‹ m 2 › for iron pnictides are much less than that of the insulating alkaline iron selenides, there must be significant hybridization of Fe 3 d with pnictide p orbitals and, among themselves, in iron pnictides, which leads to a metallic state where the Hund's coupling is less important than in the atomic limit [36] . This is consistent with the fact that a pure Heisenberg Hamiltonian cannot describe the entire spin wave spectra in AF iron pnictides [24] , [25] , [26] and iron chalcogenide Fe 1.05 Te (ref. 27 ). It is instructive to compare the effective magnetic exchange couplings in different AF parent compounds of iron-based superconductors. First, comparing Rb 0.89 Fe 1.58 Se 2 with Fe 1.05 Te (ref. 27 ), we note that, although their static AF orders have completely different structures, these two iron chalcogenides are very similar in terms of the values of their effective exchange couplings. Both of them have, first, large FM J 1 (or J 1 a ); second, large anisotropy between the two NN couplings J 1 ( J 1 a ) and J′ 1 (or J 1 b ); and, third, AF NNN couplings and small anisotropy between two NNN couplings J 2 (or, J 2 a ) and J′ 2 (or J 2b ). Finally, there are significant AF–NNNN couplings J 3 . Therefore, the presence of the iron vacancy ordering in Rb 0.89 Fe 1.58 Se 2 reduces magnetic frustration and stabilizes the block AF structure, but does not change the local magnetic exchange coupling strengths as compared with Fe 1.05 Te, even though the 5 p orbitals of Te should be larger than the 4 p orbitals of Se. Second, comparing Rb 0.89 Fe 1.58 Se 2 to iron-pnictides, we find that there are important differences as well as essential common features: the differences include the large differences in the sum of the fluctuating local moments ‹ m 2 › and the NN exchange couplings. However, the NNN exchange couplings are rather similar in spite of their insulating and metallic ground states. To summarize, whereas the NN exchange couplings vary significantly according to the spin configurations between the corresponding two NN sites in the magnetically ordered states of alkaline iron selenides, iron tellurides, and iron pnictides, the AF–NNN exchange coupling remains almost uniform for these materials. This is consistent with the idea that the NNN coupling J 2 is mainly determined by a local superexchange mechanism mediated by As or Se/Te (ref. 37 ). Therefore, regardless of their metallic or insulating ground states, different AF structures and Néel temperatures, spin waves in all parent compounds of Fe-based superconductors have a similar energy scale with a common NNN magnetic coupling controlled by the local superexchange interactions. As superconductivity in Fe-based materials arises from electron or hole-doping of their AF parent compounds, the similarities in the magnetic properties of parent compounds suggest that the microscopic origin of superconductivity for doped superconductors should be similar as well. Single-crystal Rb 0.89 Fe 1.58 Se 2 Our single crystals of Rb y Fe 1.6+ x Se 2 were grown using flux method. High-purity Fe, Se and Rb were mixed in appropriate stoichiometry and placed inside an alumina crucible. The crucible was sealed in Ar-filled silica ampoule. The mixture was heated to 950 °C for 5 h followed by 5 °C per hr cooling down to 900 °C, and then furnace cooling down to room temperature [11] . The actual crystal composition of Rb 0.89 Fe 1.58 Se 2 was determined inductively coupled plasma analysis. Extra spin wave data In addition to the time-of-flight measurements presented in Figures 1 , 2 , 3 , 4 , we have taken triple-axis spectrometer measurements on HB-1 at High Flux isotope reactor, Oak Ridge National Laboratory, to determine the low-energy spin-anisotropy gap. Before showing the results, we note that, although the scattering cross-section is related to the dynamic structure factor S ( Q,E ), it is proportional to the imaginary part of the dynamic susceptibility χ″ ( Q,ω ) if the temperature is much lower than the lowest energy spin waves. Theoretically, one has S ( Q,E )=1/(1−exp(− E /( k B T ))) χ″ ( Q,E ). If k B T « E , as is the case of the experiment, one has S ( Q,E ) χ″ ( Q,E ). 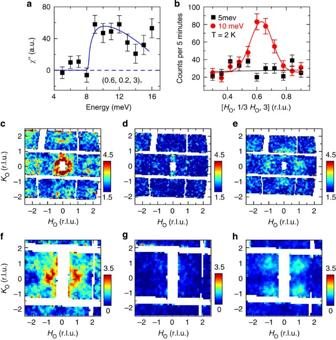Figure 5: Triple-axis spectrometer data and extra spin wave images near spin gaps on Rb0.89Fe1.58Se2. (a) Constant-Qscan at the AF wave vectorQAF=(0.6,0.2,3) r.l.u. with background subtracted, and corrected for Bose population factor. There is a clear spin gap belowE=8 meV. The data were collected on HB-1 triple-axis spectrometer. (b) Constant-energy scans across the AF wave vector atE=5 meV andE=10 meV. The data confirm the presence of a spin gap at 5 meV. The vertical error bars indicate the statistical errors of one standard deviation. Spin wave images in the (Ho,Ko) plane for energy transfers of (c)E=74±4; (d) 82±4;(e) 90±4; (f) 140±10; (g) 155±15; (h) 195±15 meV. There are clearly no spin wave excitations atE=82±4 and 155±15 meV. Figure 5a shows χ″ ( Q,E ) at Q AF =(0.6,0.2,3), which clearly establishes the anisotropy spin gap of ~8 meV. Constant energy scans at 5 meV and 10 meV, shown in Figure 5b, confirm the presence of the spin gap below 8 meV. To further demonstrate the presence of spin gaps around 80 and 160 meV, we show, in Figure 5c–e, constant energy cuts for energies of E =74±4 meV, 82±4 meV, and 90±4 meV, respectively. There are clearly no magnetic scattering near E =82±4 meV ( Fig. 5d ). Figure 5f–h show similar constant-energy images at E =140±10, 155±15, and 195±15 meV. The scattering near E =155±15 meV are featureless, confirming the presence of a spin gap at this energy. Figure 5: Triple-axis spectrometer data and extra spin wave images near spin gaps on Rb 0.89 Fe 1.58 Se 2 . ( a ) Constant- Q scan at the AF wave vector Q AF =(0.6,0.2,3) r.l.u. with background subtracted, and corrected for Bose population factor. There is a clear spin gap below E =8 meV. The data were collected on HB-1 triple-axis spectrometer. ( b ) Constant-energy scans across the AF wave vector at E =5 meV and E =10 meV. The data confirm the presence of a spin gap at 5 meV. The vertical error bars indicate the statistical errors of one standard deviation. Spin wave images in the ( H o ,K o ) plane for energy transfers of ( c ) E =74±4; ( d ) 82±4;( e ) 90±4; ( f ) 140±10; ( g ) 155±15; ( h ) 195±15 meV. There are clearly no spin wave excitations at E =82±4 and 155±15 meV. Full size image How to cite this article: Wang, M. et al . Spin waves and magnetic exchange interactions in insulating Rb 0.89 Fe 1.58 Se 2 . Nat. Commun. 2:580 doi: 10.1038/ncomms1573 (2011).